A molecular brake controls the magnitude of long-term potentiation Overexpression of suprachiasmatic nucleus circadian oscillatory protein (SCOP), a negative ERK regulator, blocks long-term memory encoding. Inhibition of calpain-mediated SCOP degradation also prevents the formation of long-term memory, suggesting rapid SCOP breakdown is necessary for memory encoding. However, whether SCOP levels also control the magnitude of long-term synaptic plasticity is unknown. Here we show that following synaptic activity-induced SCOP degradation, SCOP is rapidly replaced via mTOR-mediated protein synthesis. We further show that early SCOP degradation is specifically catalysed by μ-calpain, whereas late SCOP resynthesis is mediated by m-calpain. We propose that μ-calpain promotes long-term potentiation induction by degrading SCOP and activating ERK, whereas m-calpain activation limits the magnitude of potentiation by terminating the ERK response via enhanced SCOP synthesis. This unique braking mechanism could account for the advantages of spaced versus massed training in the formation of long-term memory. Long-term potentiation (LTP) of glutamatergic transmission induced by brief, patterned stimulation of afferents fulfills several requirements for a high-capacity memory mechanism, including rapid induction, extreme persistence and synapse specificity [1] . Accordingly, a large amount of work has led to a detailed description of the induction, expression and stabilization phases of LTP, and the identification of key signaling cascades involved in each of these steps. In contrast, the factors that control the magnitude of LTP are still poorly understood. The present study introduces a novel set of signaling events that impose a limit on the degree of lasting potentiation produced by naturalistic induction events. Transient extracellular signal-regulated kinase (ERK) activation has been repeatedly shown to be necessary for LTP induction [2] , [3] , [4] and for triggering mammalian target of rapamycin (mTOR)-dependent local protein synthesis [3] . SCOP (suprachiasmatic nucleus circadian oscillatory protein) inhibits ERK 1/2 by binding and trapping its activator Ras in the inactive form [5] . In cultured neurons, brain-derived neurotrophic factor (BDNF) or NMDA ( N -methyl- D -aspartate) receptor activation can remove this inhibition through calpain-mediated SCOP degradation. Calpain regulation of SCOP has important functional implications, as SCOP overexpression blocked novel object recognition memory [6] , whereas calpain inhibition blocked learning-induced decrease in SCOP levels in hippocampus. We had earlier proposed that calpain activation leads to modifications of the dendritic spine cytoskeleton and a redistribution of glutamate receptors, resulting in a long-lasting changes in synapse structure and function [7] , [8] . Several lines of evidence support this hypothesis, including reports from different groups that calpain inhibitors applied before and during inducing stimulation block the subsequent development of LTP [9] , [10] , [11] . More recently, we found that BDNF, whose release after LTP induction [12] is required for stable potentiation, activates m-calpain, probably via ERK-mediated phosphorylation at serine 50 (ref. 13 ), resulting in mTOR-stimulated local protein synthesis via phosphatase and tensin homologue (PTEN) truncation [14] . This raises the possibility that mTOR activation might serve to replenish SCOP pools, thereby terminating theta-burst stimulation (TBS)-induced ERK activation. Our studies were directed at testing the idea that both degradation and synthesis of SCOP are important for LTP process, and at understanding the mechanism as well as the functional significance of the rapid return of ERK inhibition. Combined with earlier findings, the results strongly suggest that μ-calpain-mediated SCOP degradation is involved in LTP induction, whereas m-calpain-mediated stimulation of mTOR-dependent SCOP synthesis restricts the magnitude of potentiation during early consolidation. Thus, rapid activity-dependent changes in SCOP levels resulting from the dual and opposite effects of μ- and m-calpain control the formation and extent of LTP in the hippocampus. The existence of this molecular mechanism controlling the magnitude of potentiation has clear implications for our understanding of learning and memory. Reciprocal changes in SCOP and ERK following BDNF treatment Shimizu et al. [6] showed that BDNF causes a rapid decrease in SCOP levels associated with increase in ERK phosphorylation/activation in cultured neurons. We extended this result to acute hippocampal slices and found, as was observed in cultured neurons, that both effects returned to baseline levels within 40 min despite the continued presence of the neurotrophin ( Fig. 1a–c ). Pretreatment with calpain inhibitor III (CI-III; 10 μM) completely eliminated BDNF-induced decrease in SCOP levels and the concomitant increase in phosphorylated ERK (p-ERK) levels ( Fig. 1d–f ). Collectively, these results suggest that BDNF-driven calpain activation results in degradation of a negative modulator (SCOP) of ERK, as described in previous work, followed by a surprisingly rapid recovery of the modulator associated with termination of ERK activation. 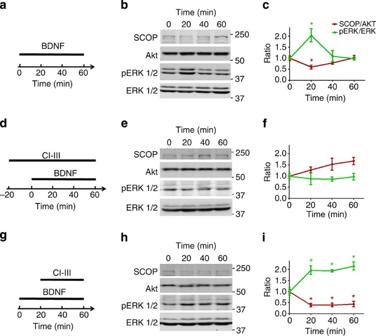Figure 1: Effects of CI-III on BDNF-induced changes in levels of SCOP and p-ERK. (a,d,g) Experimental protocols: hippocampal slices were prepared from adult rats and were treated with BDNF (100 ng ml−1) for the indicated periods of time in the absence or presence of CI-III (10 μM), as indicated. (b,e,h) Representative western blots for SCOP, Akt, p-ERK and ERK under various experimental conditions. (c,f,i) Quantitative analysis of the levels of SCOP (normalized to the values of Akt) and p-ERK/ERK ratios under various experimental conditions. In all cases, results are means±s.e.m. of three experiments. *P<0.05, as compared with time point 0, one-way analysis of variance followed by Bonferroni test. Figure 1: Effects of CI-III on BDNF-induced changes in levels of SCOP and p-ERK. ( a , d , g ) Experimental protocols: hippocampal slices were prepared from adult rats and were treated with BDNF (100 ng ml −1 ) for the indicated periods of time in the absence or presence of CI-III (10 μM), as indicated. ( b , e , h ) Representative western blots for SCOP, Akt, p-ERK and ERK under various experimental conditions. ( c , f , i ) Quantitative analysis of the levels of SCOP (normalized to the values of Akt) and p-ERK/ERK ratios under various experimental conditions. In all cases, results are means±s.e.m. of three experiments. * P <0.05, as compared with time point 0, one-way analysis of variance followed by Bonferroni test. Full size image We next asked whether calpain was involved in SCOP recovery by applying its inhibitor starting 20 min after the onset of BDNF treatment. The results were remarkable: the neurotrophin produced the expected decrease in SCOP levels with associated increase in ERK activation, but these effects continued throughout the remainder of the 1-h incubation period, and ERK recovery was eliminated ( Fig. 1g–i ). We recently reported that calpain degrades PTEN, an inhibitor of mTOR-mediated protein synthesis [14] , raising the possibility that BDNF-induced activation of the protease results in accelerated synthesis of replacement copies of SCOP. In support of this idea, when BDNF treatment of hippocampal slices was performed in the presence of cycloheximide, a general protein synthesis inhibitor, or rapamycin, an inhibitor of mTOR-mediated protein synthesis, the recovery of SCOP levels was prevented and p-ERK levels remained elevated above control levels ( Fig. 2a–f ). To further confirm that BDNF promotes de novo SCOP synthesis, we performed pulse-chase experiments in cortical synaptoneurosomes using a modified amino acid, L -azidohomoalanine, which is incorporated into newly synthesized proteins and can later be labelled with biotin. Total SCOP was immunoprecipitated after metabolic labelling of nascent proteins. Newly synthesized (biotin labelled) and total SCOP were then detected, using infrared dye-conjugated Streptavidin and anti-SCOP antibody, respectively. Treatment of synaptoneurosomes with BDNF for 60 min significantly increased the levels of newly synthesized SCOP as compared with control, an effect that was absent in synaptoneurosomes pretreated with rapamycin ( Fig. 2g–i ). This result further confirms the hypothesis proposed by Shimizu et al. [6] that balance between degradation and synthesis is responsible for the dual effect of BDNF on SCOP levels and ERK activation. 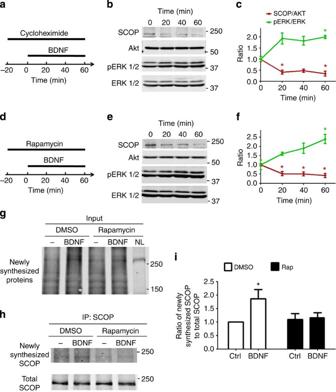Figure 2: Effects of cycloheximide and rapamycin on BDNF-induced changes in levels of SCOP and p-ERK. (a,d) Experimental design: hippocampal slices were treated with BDNF (100 ng ml−1) for the indicated periods of time in the presence of cycloheximide (25 μM) or rapamycin (1 μM). (b,e) Representative western blottings for SCOP, Akt, p-ERK and ERK under various experimental conditions. (c,f) Quantitative analysis of the levels of SCOP (normalized to the values of Akt) and p-ERK/ERK ratios under various experimental conditions. In all cases, results are means±s.e.m. of three experiments. *P<0.05, as compared with time point 0, one-way analysis of variance (ANOVA) followed by Bonferroni test. (g) Representative blot for all newly synthesized (biotin labelled) proteins larger than 150 kDa from synaptoneurosomes before immunoprecipitation (input) as detected by IRDye 800CW Streptavidin. Note that the second lane (BDNF-treated sample) shows denser labelling than the other lanes. NL (not labelled) line is from naive synaptoneurosomes without metabolic labelling (negative control). (h) Representative western blottings for newly synthesized (biotin labelled) and total SCOP, after treatment of cortical synaptoneurosomes with BDNF (100 ng ml−1) in the absence or presence of rapamycin (1 μM), and subsequent immunoprecipitation with SCOP antibody. (i) Quantitative analysis of the levels of newly synthesized SCOP (normalized to total SCOP). Data are means±s.e.m. of four experiments. *P<0.05, as compared with control, two-way ANOVA followed by Bonferroni test. Figure 2: Effects of cycloheximide and rapamycin on BDNF-induced changes in levels of SCOP and p-ERK. ( a , d ) Experimental design: hippocampal slices were treated with BDNF (100 ng ml −1 ) for the indicated periods of time in the presence of cycloheximide (25 μM) or rapamycin (1 μM). ( b , e ) Representative western blottings for SCOP, Akt, p-ERK and ERK under various experimental conditions. ( c , f ) Quantitative analysis of the levels of SCOP (normalized to the values of Akt) and p-ERK/ERK ratios under various experimental conditions. In all cases, results are means±s.e.m. of three experiments. * P <0.05, as compared with time point 0, one-way analysis of variance (ANOVA) followed by Bonferroni test. ( g ) Representative blot for all newly synthesized (biotin labelled) proteins larger than 150 kDa from synaptoneurosomes before immunoprecipitation (input) as detected by IRDye 800CW Streptavidin. Note that the second lane (BDNF-treated sample) shows denser labelling than the other lanes. NL (not labelled) line is from naive synaptoneurosomes without metabolic labelling (negative control). ( h ) Representative western blottings for newly synthesized (biotin labelled) and total SCOP, after treatment of cortical synaptoneurosomes with BDNF (100 ng ml −1 ) in the absence or presence of rapamycin (1 μM), and subsequent immunoprecipitation with SCOP antibody. ( i ) Quantitative analysis of the levels of newly synthesized SCOP (normalized to total SCOP). Data are means±s.e.m. of four experiments. * P <0.05, as compared with control, two-way ANOVA followed by Bonferroni test. Full size image SCOP decrease mediates transient ERK activation in LTP To directly test whether calpain regulates SCOP levels and subsequently ERK activity during LTP, we repeated the above experiments using TBS stimulation of hippocampal CA1 minislices from adult rats. SCOP levels, as assessed with immunoblottings, were significantly reduced 8 min after TBS stimulation in CA1 minislices, but returned to control levels 50 min after TBS. As in BDNF-treated hippocampal slices, p-ERK levels followed a reciprocal pattern: a marked elevation when SCOP levels were decreased and a delayed return to baseline as SCOP subsequently returned to control values ( Fig. 3a–c ). Pretreatment of slices with CI-III eliminated TBS-induced decrease in SCOP levels and the associated increase in ERK activation ( Fig. 3d–f ). However, when CI-III (10 μM) was applied after TBS application, SCOP levels remained decreased, and correspondingly p-ERK levels remained elevated ( Fig. 3g–j ). Similar results were obtained when using tetraethylammonium (TEA)-induced chemical LTP [15] , [16] , [17] in rat acute hippocampal slices ( Supplementary Fig. 1 ). These findings suggested that SCOP is rapidly synthesized following its degradation stimulated by increased neuronal activity. Under basal conditions, cycloheximide treatment of cortical synaptoneurosomes decreased SCOP levels with a t1/2 of ~90 min, suggesting that SCOP turns over rapidly and is replenished by protein synthesis ( Supplementary Fig. 2a ). Consistently, ERK phosphorylation gradually increased over time after treatment with cycloheximide ( Supplementary Fig. 2b ). The results obtained with BDNF, TBS or TEA lead to the conclusion that LTP is associated with rapid degradation and recovery of SCOP, resulting in a pronounced but transient stimulation of ERK, consistent with previous study showing that TBS stimulation causes a rapid, short-lived increase in ERK phosphorylation in CA3–CA1 synapses of hippocampal slices [18] . Calpain appears to be involved in both the loss and recovery of SCOP, and thus in the initiation and then the termination of ERK activation. 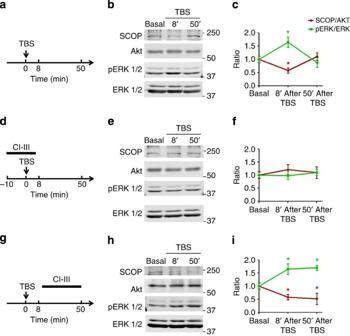Figure 3: Effects of calpain inhibition on TBS-induced changes in adult hippocampal CA1 minislices. (a,d,g) Experimental protocol: hippocampal CA1 minislices were prepared from adult rats and were stimulated by TBS in the absence or presence of CI-III (10 μM), as indicated. (b,e,h) Representative western blottings for SCOP, Akt, p-ERK and ERK under various experimental conditions. (c,f,i) Quantitative analysis of the levels of SCOP (normalized to the values of Akt) and p-ERK/ERK ratios under various experimental conditions. Results are means±s.e.m. of three to eight experiments. *P<0.05, as compared with time point 0, one-way analysis of variance followed by Bonferroni test. Figure 3: Effects of calpain inhibition on TBS-induced changes in adult hippocampal CA1 minislices. ( a , d , g ) Experimental protocol: hippocampal CA1 minislices were prepared from adult rats and were stimulated by TBS in the absence or presence of CI-III (10 μM), as indicated. ( b , e , h ) Representative western blottings for SCOP, Akt, p-ERK and ERK under various experimental conditions. ( c , f , i ) Quantitative analysis of the levels of SCOP (normalized to the values of Akt) and p-ERK/ERK ratios under various experimental conditions. Results are means±s.e.m. of three to eight experiments. * P <0.05, as compared with time point 0, one-way analysis of variance followed by Bonferroni test. Full size image We then used immunohistochemistry to verify whether calpain inhibition before TBS could block ERK activation, while the same treatment applied after TBS could prolong ERK phosphorylation in dendritic spines. A single train of ten theta bursts was applied to the Schaffer-commissural pathway in field CA1b of hippocampus and slices were collected at various times post TBS. Sectioning and immunostaining with antibodies selective for p-ERK were performed as described in Methods. A marked increase in p-ERK labelling of spines and dendrites was observed at 5 min post TBS in the apical dendritic field adjacent to the stimulation site, an effect that was altogether absent in zones outside the Schaffer-commissural termination field. The increased labelling was, as expected from the literature, absent in slices collected 50 min after TBS ( Fig. 4 ). CI-III applied before TBS partially but significantly blocked ERK activation at 5 min after TBS ( Fig. 4 ). In contrast, when slices were treated with CI-III starting 10 min after TBS, a large number of dendrites and spines in the vicinity of the stimulating electrode were still p-ERK immunopositive at 50 min post TBS ( Fig. 4 ), an effect that was highly significant relative to TBS alone. 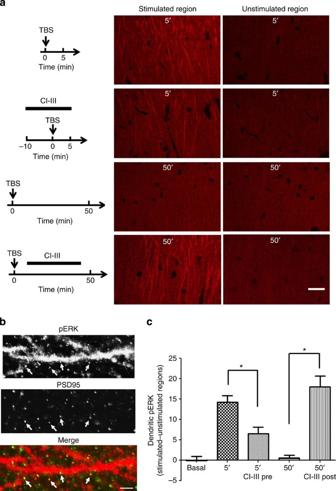Figure 4: TBS-induced ERK activation is differentially affected by pre- or post-TBS CI-III treatment. Hippocampal slices were prepared from adult rats and subjected to various experimental conditions. At the indicated times, slices were fixed, re-sectioned and processed for immunohistochemistry for p-ERK. Images of stimulated and unstimulated regions from two most representative sections of each slice were chosen for analysis. (a) Representative images. Top: p-ERK immunoreactivity at 5 min after TBS (10 bursts of 4 pulses (100 Hz) delivered at 5 Hz) in slices treated with vehicle or CI-III (10 μM) for 10 min before and continued for 5 min after TBS. Bottom: p-ERK immunoreactivity at 50 min after TBS in slices treated with vehicle or CI-III (10 μM) for 30 min starting 10 min after TBS. Scale bar, 20 μm. (b) High-magnification images of dendrites in stimulated region double-stained with p-ERK and PSD-95 antibodies, showing the co-localization of p-ERK and PSD-95 (arrows). Scale bar, 2 μm. (c) Quantitative analysis of p-ERK immunostaining. The average p-ERK intensity was determined in a 120 × 60 μm2area in the dendritic field of CA1. Image intensities from stimulated regions were subtracted from those of unstimulated regions of the same slice to correct for slice-to-slice variation in staining intensity, as described inref.38. Shown are means±s.e.m. ofn=8. *P<0.01, one-way analysis of variance followed by Bonferroni test. Figure 4: TBS-induced ERK activation is differentially affected by pre- or post-TBS CI-III treatment. Hippocampal slices were prepared from adult rats and subjected to various experimental conditions. At the indicated times, slices were fixed, re-sectioned and processed for immunohistochemistry for p-ERK. Images of stimulated and unstimulated regions from two most representative sections of each slice were chosen for analysis. ( a ) Representative images. Top: p-ERK immunoreactivity at 5 min after TBS (10 bursts of 4 pulses (100 Hz) delivered at 5 Hz) in slices treated with vehicle or CI-III (10 μM) for 10 min before and continued for 5 min after TBS. Bottom: p-ERK immunoreactivity at 50 min after TBS in slices treated with vehicle or CI-III (10 μM) for 30 min starting 10 min after TBS. Scale bar, 20 μm. ( b ) High-magnification images of dendrites in stimulated region double-stained with p-ERK and PSD-95 antibodies, showing the co-localization of p-ERK and PSD-95 (arrows). Scale bar, 2 μm. ( c ) Quantitative analysis of p-ERK immunostaining. The average p-ERK intensity was determined in a 120 × 60 μm 2 area in the dendritic field of CA1. Image intensities from stimulated regions were subtracted from those of unstimulated regions of the same slice to correct for slice-to-slice variation in staining intensity, as described inref. [38] . Shown are means±s.e.m. of n =8. * P <0.01, one-way analysis of variance followed by Bonferroni test. Full size image Calpain activity after TBS restricts the magnitude of LTP What, if any, are the physiological consequences of blocking SCOP recovery and prolonging ERK activation following LTP induction? We began answering this question by first repeating prior work on the effects of calpain inhibition on the induction, expression and rapid consolidation of LTP. Infusion of CI-III (10 μM) starting 10 min before TBS had no evident effects on baseline or on the initial expression of LTP but, in agreement with previous reports [10] , [11] , completely blocked the subsequent stabilization of the potentiation effect ( Fig. 5a ). Notably, it also caused no detectable changes in the burst responses during TBS ( Supplementary Fig. 3 ), indicating that calpain inhibition did not interfere with frequency facilitation or NMDA receptor function. We also reproduced a previous finding that application of CI-III 1 h after TBS did not modify established LTP ( Fig. 5a ) [10] . Remarkably, infusion of CI-III starting 10 min after TBS produced an unexpected result: the slope of the already potentiated responses rapidly increased and, over the next 30 min, reached values more than twice as large as those normally found 1 h after a single train of theta bursts ( Fig. 5a,b ). Similar results were obtained with CI-IV ( Supplementary Fig. 4 ), which is reported to have a different pattern of inhibition for cysteine proteases than CI-III [19] . 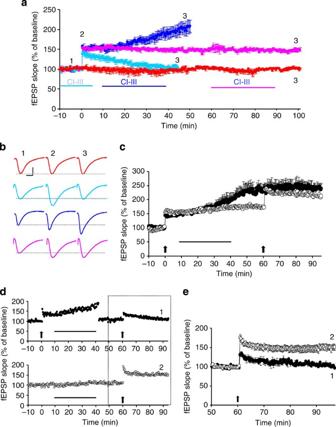Figure 5: Effects of calpain inhibition at various times before or after LTP induction. (a) Time-dependent effects of calpain inhibition on LTP. Hippocampal slices were prepared from adult rats and LTP was induced in field CA1 by TBS (black arrow). Vehicle or CI-III (10 μM) was applied for 10 min before and continued 5 min after TBS (cyan). Alternatively, CI-III (10 μM) was applied for 30 min starting 10 min (blue) or 60 min (magenta) post TBS. Slopes of field excitatory postsynaptic potentials (fEPSPs) are expressed as per cent of the average values recorded during the 10-min baseline (means±s.e.m. of five to ten slices from three to five animals). Basal synaptic transmission did not change during the recording period (red). (b) Representative traces for fEPSPs recorded at the indicated time points (1, 2 and 3) under different experimental conditions. Calibration: 0.5 mV per 5 ms. (c) Post-TBS calpain inhibition blocks TBS2-induced further potentiation. TBS was applied as indicated by arrows. CI-III (10 μM) was applied during the time indicated by the horizontal lines. A second TBS was delivered 60 min after the first TBS and fEPSP was recorded for an additional 40 min (means±s.e.m. of six to eight slices from three to four animals). (d) Top: CI-III (10 μM) was applied for 30 min starting 10 min after TBS1 (arrow). At the end of calpain inhibitor treatment, stimulation intensity was decreased to obtain a response equivalent to the pre-TBS value. After 20 min, TBS2 was delivered and responses recorded for an additional 40 min (representative experiment). Bottom: CI-III (10 μM) was applied to naive slices for 30 min. After 20 min, TBS was applied and responses recorded for an additional 40 min (representative experiment). (e) Comparison of the responses highlighted ind(means±s.e.m. of six to eight slices). Figure 5: Effects of calpain inhibition at various times before or after LTP induction. ( a ) Time-dependent effects of calpain inhibition on LTP. Hippocampal slices were prepared from adult rats and LTP was induced in field CA1 by TBS (black arrow). Vehicle or CI-III (10 μM) was applied for 10 min before and continued 5 min after TBS (cyan). Alternatively, CI-III (10 μM) was applied for 30 min starting 10 min (blue) or 60 min (magenta) post TBS. Slopes of field excitatory postsynaptic potentials (fEPSPs) are expressed as per cent of the average values recorded during the 10-min baseline (means±s.e.m. of five to ten slices from three to five animals). Basal synaptic transmission did not change during the recording period (red). ( b ) Representative traces for fEPSPs recorded at the indicated time points (1, 2 and 3) under different experimental conditions. Calibration: 0.5 mV per 5 ms. ( c ) Post-TBS calpain inhibition blocks TBS2-induced further potentiation. TBS was applied as indicated by arrows. CI-III (10 μM) was applied during the time indicated by the horizontal lines. A second TBS was delivered 60 min after the first TBS and fEPSP was recorded for an additional 40 min (means±s.e.m. of six to eight slices from three to four animals). ( d ) Top: CI-III (10 μM) was applied for 30 min starting 10 min after TBS1 (arrow). At the end of calpain inhibitor treatment, stimulation intensity was decreased to obtain a response equivalent to the pre-TBS value. After 20 min, TBS2 was delivered and responses recorded for an additional 40 min (representative experiment). Bottom: CI-III (10 μM) was applied to naive slices for 30 min. After 20 min, TBS was applied and responses recorded for an additional 40 min (representative experiment). ( e ) Comparison of the responses highlighted in d (means±s.e.m. of six to eight slices). Full size image Recent work showed that delivery of a second TBS bout (‘TBS2’) after a 1-h delay more than doubles the magnitude of LTP produced by TBS1 (refs 20 , 21 , 22 ) and that the enhancement is likely to be due to recruitment of additional synapses into the potentiated state [22] . We confirmed the ‘LTP2’ effect in the present studies, and found that its magnitude is about the same as that produced by delayed application of CI-III ( Fig. 5c , open circles). These observations raise the possibility that post-TBS infusion of a calpain inhibitor, acting via increase in p-ERK, unmasks a latent potentiation produced by TBS1 in a large population of synapses. If so, then the novel enhancement phenomenon described here should occlude the LTP2 effect. To test this hypothesis, we first confirmed that the enhanced LTP remained in place following a 20-min washout of the calpain inhibitor ( Fig. 5c ) and that normal LTP could be induced in a ‘naive’ pathway at this time point ( Fig. 5d , top). TBS2 delivered after washout, and 1 h after TBS1, had no further effect on the magnitude of LTP ( Fig. 5c , closed circles). To confirm that the absence of additional LTP was due to the saturation of synaptic potentiation but not to a ceiling effect on evoked synaptic responses, we decreased the intensity of stimulation to generate responses of the same magnitude as during baseline, before delivering the second TBS. Again, no evidence for LTP2 was found ( Fig. 5d , bottom; also see Fig. 5e ). To further test the selectivity of the effect of calpain inhibitor on stimulated synapses, we used a second stimulation electrode (S2), which was placed on the opposite side of the recording electrode from the first stimulation electrode (S1; Supplementary Fig. 5a ). In the S1 pathway, TBS-induced LTP and CI-III (10 μM) applied 10 min post TBS elicited further potentiation. However, responses in the control pathway (S2) remained unchanged in the absence or presence of CI-III ( Supplementary Fig. 5b ). These data indicated that CI-III only had effects on TBS-stimulated synapses. ERK inactivation after TBS is necessary for LTP restriction We then tested the hypothesis that SCOP degradation and the resulting ERK activation were involved in the LTP enhancement effect of post-TBS calpain inhibition by applying two different inhibitors of mitogen-activated protein kinase (MEK), U0126 (5 μM) or PD98059 (5 μM), alone or in the presence of CI-III (10 μM) 10 min after TBS. Both inhibitors completely prevented the enhancing effect of CI-III on LTP ( Fig. 6a,b ). Application of the MEK inhibitors alone at this concentration had no effect on LTP consolidation, a result consistent with a previous report that ERK activation is not required for LTP consolidation [23] . Quantitative analysis of the results indicated that the effects of CI-III on LTP and the blocking effects of both U0126 and PD98059 were highly statistically significant, as compared with TBS alone ( Fig. 6d ). As our results indicated that SCOP synthesis was responsible for the late phase of ERK inhibition induced by BDNF treatment or TBS stimulation, we also tested the effects of rapamycin applied 10 min after TBS. Interestingly, application of rapamycin shortly after TBS caused a progressive enhancement of LTP, similar to that produced by post-TBS application of CI-III ( Fig. 6c,d ). Similar to rapamycin, a 10-min post-TBS application of cycloheximide, a general protein synthesis inhibitor, further enhanced the magnitude of LTP ( Supplementary Fig. 6 ). 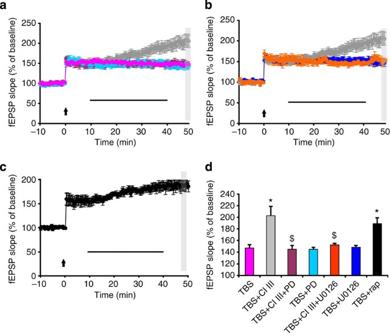Figure 6: ERK inhibition prevents and mTOR inhibition mimics calpain inhibition-induced LTP enhancement. Hippocampal slices were prepared from adult rats and LTP was induced by TBS as inFig. 1. The MEK inhibitors PD98059 (5 μM) (a) or U0126 (5 μM) (b) were applied together with CI-III (10 μM) for 30 min. The data for the grey symbols inaandb, which were used as the reference, are fromFig. 5a(blue symbol). In all cases, the slopes of the field excitatory postsynaptic potentials (fEPSPs) are expressed as per cent of the average values recorded during the 10-min baseline, and are means±s.e.m. of five to ten slices prepared from three to five animals. (c) Effects of rapamycin (1 μM) applied for 30 min (horizontal bar) starting at 10 min after TBS on hippocampal LTP. (d) Summary of the amplitude of LTP measured within the grey area corresponding to 49–50 min after TBS (note that the data for TBS and TBS+CI-III are fromFig. 5a). *P<0.01, as compared with TBS alone;§P<0.01, as compared with TBS+CI-III (one-way analysis of variance followed by Bonferroni test). The slopes of the fEPSPs are expressed as per cent of the average values recorded during the 10-min baseline, and are means±s.e.m. of five to ten slices prepared from three to five animals. Figure 6: ERK inhibition prevents and mTOR inhibition mimics calpain inhibition-induced LTP enhancement. Hippocampal slices were prepared from adult rats and LTP was induced by TBS as in Fig. 1 . The MEK inhibitors PD98059 (5 μM) ( a ) or U0126 (5 μM) ( b ) were applied together with CI-III (10 μM) for 30 min. The data for the grey symbols in a and b , which were used as the reference, are from Fig. 5a (blue symbol). In all cases, the slopes of the field excitatory postsynaptic potentials (fEPSPs) are expressed as per cent of the average values recorded during the 10-min baseline, and are means±s.e.m. of five to ten slices prepared from three to five animals. ( c ) Effects of rapamycin (1 μM) applied for 30 min (horizontal bar) starting at 10 min after TBS on hippocampal LTP. ( d ) Summary of the amplitude of LTP measured within the grey area corresponding to 49–50 min after TBS (note that the data for TBS and TBS+CI-III are from Fig. 5a ). * P <0.01, as compared with TBS alone; § P <0.01, as compared with TBS+CI-III (one-way analysis of variance followed by Bonferroni test). The slopes of the fEPSPs are expressed as per cent of the average values recorded during the 10-min baseline, and are means±s.e.m. of five to ten slices prepared from three to five animals. Full size image m-Calpain activation limits the magnitude of LTP Two major isoforms of calpain are present in the brain, μ- and m-calpain, which differ by their calcium requirements for activation in in vitro assays, with μ-calpain requiring micromolar and m-calpain requiring millimolar calcium concentration for activation. As we previously showed that BDNF stimulated m-calpain through ERK-mediated phosphorylation [13] , and that m-calpain-dependent PTEN degradation was involved in BDNF-mediated mTOR stimulation and stimulation of local protein synthesis [14] , we postulated that m-calpain activation could be responsible for the changes in SCOP metabolism following TBS. We tested the effects of a dipeptide ketoamide, Z-Leu-Abu-CONH-CH 2 -C 6 H 3 (3,5-(OMe) 2 ) (mCalp-I), which has been reported to have a Ki of 22 nM against m-calpain versus a Ki of 2.3 μM against μ-calpain [24] . We first verified that mCalp-I was indeed more selective for m- than for μ-calpain, by determining its half maximal inhibitory concentration (IC 50 ) for purified m-calpain- or μ-calpain-induced degradation of Succinyl-Leu-Tyr-7-amino-4-methylcoumarin (Suc-Leu-Tyr-AMC; Supplementary Fig. 7 ). From the IC 50 , we used the Cheng–Prusoff equation to determine the Kis of mCalp-I for m- and μ-calpain; in our hand, the Ki for m-calpain was 25 nM and for μ-calpain 0.94 μM, in close agreement with the reported values. We then tested the effects of mCalp-I on TEA-mediated SCOP and PTEN degradation ( Fig. 7a–f ). Interestingly, mCalp-I (200 nM) did not prevent TEA-mediated SCOP degradation when added before TEA but it prevented its recovery during prolonged incubation ( Fig. 7d–f ). On the other hand, mCalp-I did prevent TEA-mediated PTEN degradation, further suggesting that m-calpain activation is responsible for TEA-mediated PTEN degradation and stimulation of SCOP synthesis. Application of mCalp-I before TBS did not affect LTP induction ( Fig. 7g,h ); however, it did produce the same enhancement of LTP starting about 15 min after TBS ( Fig. 7g,h ). It also enhanced LTP when applied 20 min after TBS ( Fig. 7g,h ). 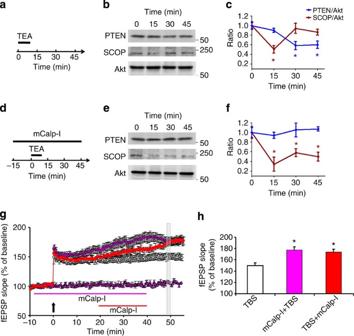Figure 7: Effects of an m-calpain-specific inhibitor on TEA-mediated SCOP and PTEN degradation and on LTP. (a–f) Hippocampal slices were prepared from adult rats and were treated with TEA (20 mM) for 10 min, and collected at the indicated times. TEA and mCalp-I (200 nM) were applied as shown inaandd. (bande) Representative western blottings for SCOP, PTEN and Akt at the indicated times. (c,f) Quantitative analysis of the levels of SCOP and PTEN (normalized to the values of Akt). In all cases, results are means±s.e.m. of three experiments. *P<0.05, as compared with time point 0, one-way analysis of variance followed by Bonferroni test. (g,h) Effects of mCalp-I on TBS-induced LTP. mCalp-I (200 nM) was applied either before TBS (vertical arrow; blue circles) or 20 min after TBS (red circles). mCalp-I alone had no effect on baseline responses (blue triangles). (h) Summary of the amplitude of LTP measured within the grey area corresponding to 49–50 min after TBS. *P<0.01, as compared with TBS alone. Figure 7: Effects of an m-calpain-specific inhibitor on TEA-mediated SCOP and PTEN degradation and on LTP. ( a – f ) Hippocampal slices were prepared from adult rats and were treated with TEA (20 mM) for 10 min, and collected at the indicated times. TEA and mCalp-I (200 nM) were applied as shown in a and d . ( b and e ) Representative western blottings for SCOP, PTEN and Akt at the indicated times. ( c , f ) Quantitative analysis of the levels of SCOP and PTEN (normalized to the values of Akt). In all cases, results are means±s.e.m. of three experiments. * P <0.05, as compared with time point 0, one-way analysis of variance followed by Bonferroni test. ( g , h ) Effects of mCalp-I on TBS-induced LTP. mCalp-I (200 nM) was applied either before TBS (vertical arrow; blue circles) or 20 min after TBS (red circles). mCalp-I alone had no effect on baseline responses (blue triangles). ( h ) Summary of the amplitude of LTP measured within the grey area corresponding to 49–50 min after TBS. * P <0.01, as compared with TBS alone. Full size image The results described here constitute the first evidence that an active process regulates the magnitude of LTP in minutes to hours following the inducing stimulus. Not surprisingly, the pertinent mechanisms incorporate many novel features, including a time of action that continues for a considerable period after induction of the potentiation effect. It thus appears that theta burst stimulation both enhances synaptic responses and triggers previously undetected processes that set limits on the degree of potentiation. The present findings point to the serial activation of two isoforms of the protease calpain, both targeting a negative regulator of ERK, as being critically involved in the LTP induction/capping sequence. This collection of new phenomenology is logically related to recently reported LTP timing rules and thereby to particular aspects of learning. Below, we consider the complex cellular events uncovered in our studies before turning to these functional implications. Our results indicate that the metabolism of SCOP, a protein exhibiting a circadian rhythm in the suprachiasmatic nucleus, is subjected to rapid, activity-dependent changes, and that these lead to a critical role in regulating the timing and extent of synaptic plasticity in the hippocampus. As previously reported [6] , SCOP is rapidly degraded by calpain following BDNF treatment of hippocampal slices; it is also rapidly degraded following TBS- or TEA-induced LTP in CA1. Under all these conditions, SCOP levels rapidly recover through mTOR-mediated protein synthesis, an event that is blocked by delayed treatment with a calpain inhibitor. Our results indicate that this is due to de novo SCOP synthesis, and not to some indirect effect producing masking/unmasking epitopes of SCOP. A previous study has identified SCOP messenger RNA among the numerous mRNAs present in the neuropil of hippocampal CA1 region [25] , indicating that SCOP is likely to be synthesized locally as a result of mTOR activation. In accord with this, we recently showed that stimulation of the mTOR pathway and local protein synthesis by BDNF is due, at least in part, to m-calpain-mediated PTEN truncation [14] . Calpain activation at different time points can thus account for both the loss and recovery of SCOP following BDNF treatment, TBS- or TEA-induced potentiation. SCOP suppresses ERK and, as expected from this, changes in activation/phosphorylation of the kinase, which plays a critical role in LTP, occurred in parallel with the above-described fluctuations in levels of the negative regulator. Thus, the present results indicate that SCOP is one of the growing list of plasticity-related proteins (for example, Arc, CamKII and, possibly, various glutamate receptor subunits [26] ) that are rapidly degraded and synthesized in dendrites as a result of increased neuronal activity. Studies using various inhibitors have indicated that calpain activation is a necessary step in LTP induction. Moreover, downregulation of calpain activity through knockout of calpain-4, the small calpain subunit common to both μ-calpain and m-calpain, similarly impairs LTP [27] . As ERK activation is a necessary early step for LTP induction [2] , [3] , [4] , [23] , calpain could exert its effects on LTP induction via SCOP degradation. We confirmed the necessary prediction from this hypothesis that pretreatment of slices with a calpain inhibitor prevented SCOP degradation and the ERK activation that normally occurs with induction of LTP by theta bursts. The question then arose of what, if any, role calpain-mediated recovery of SCOP plays following the induction and initial expression of LTP. We investigated this by infusing a calpain inhibitor minutes after delivering a train of theta bursts. This led to a marked increase in the magnitude of synaptic potentiation. We therefore propose that the suppression of ERK activity by calpain-mediated increase in SCOP synthesis in the post-induction period serves to prevent the further growth of LTP. The dual role of calpain in SCOP metabolism raised the question of whether the two major isoforms of the protease (‘μ’ and ‘m’) are differentially involved in degradation versus enhanced synthesis of SCOP. Results obtained with a specific inhibitor implicated m-calpain in mTOR-dependent SCOP synthesis following induction and strongly suggested that μ-calpain is involved in SCOP degradation during the initial phase of LTP production. The differential effects of μ- and m-calpain on SCOP could be due to a different subcellular localization of the proteases. In particular, a fraction of SCOP has been shown to be present in membrane rafts, and this fraction could be degraded following NMDA receptor channel opening and the resulting μ-calpain activation [28] . On the other hand, m-calpain might be present in a different subcellular compartment at the base of dendritic spines where local dendritic protein synthesis is taking place. Thus, the biphasic effect of TBS on ERK activation, initial activation followed by delayed prevention of activation could reflect the sequential activation of μ- and m-calpain following TBS, as well as their opposite effects on SCOP levels and ERK activation ( Fig. 8 ). An alternative hypothesis is suggested by the recent discovery that BDNF promotes m-calpain activation via phosphorylation. Release of the neurotrophin during theta burst stimulation, as evidenced by activation of its TrkB receptor within synapses, is known to facilitate the cytoskeletal changes required for LTP consolidation. However, its effects on m-calpain suggest that it also engages ERK suppression machinery shown here to place limits on the magnitude of the LTP produced by those changes. 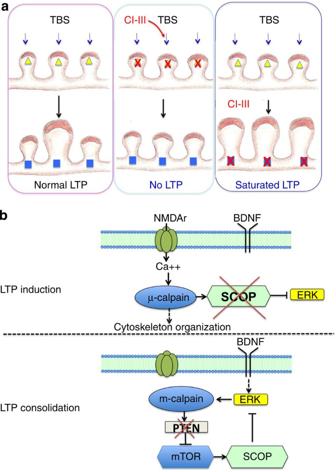Figure 8: Schematic representation of the functions of μ- and m-calpain in LTP induction and consolidation. (a) μ-Calpain activation is necessary for synaptic potentiation during LTP induction and its inhibition prevents LTP (middle panel). m-Calpain activation during consolidation limits the extent of synaptic potentiation and its inhibition results in enhanced LTP (right panel). μ-Calpain activation is indicated by yellow triangles and m-calpain by blue squares. CI-III application is indicated by red arrows. Note that we also postulate that μ-calpain and m-calpain are differentially localized in synapses. (b) Signalling pathways downstream of μ- and m-calpain in LTP induction and consolidation. In LTP induction, μ-calpain activation, possibly resulting from Ca2+influx through the NMDA receptors, results in SCOP truncation followed by ERK activation. In the consolidation period, m-calpain activation, possibly resulting from BDNF-mediated ERK activation13, stimulates mTOR-dependent protein synthesis through calpain-mediated PTEN degradation14, and in particular SCOP synthesis, which would restore normal SCOP levels, thereby preventing ERK activation. Figure 8: Schematic representation of the functions of μ- and m-calpain in LTP induction and consolidation. ( a ) μ-Calpain activation is necessary for synaptic potentiation during LTP induction and its inhibition prevents LTP (middle panel). m-Calpain activation during consolidation limits the extent of synaptic potentiation and its inhibition results in enhanced LTP (right panel). μ-Calpain activation is indicated by yellow triangles and m-calpain by blue squares. CI-III application is indicated by red arrows. Note that we also postulate that μ-calpain and m-calpain are differentially localized in synapses. ( b ) Signalling pathways downstream of μ- and m-calpain in LTP induction and consolidation. In LTP induction, μ-calpain activation, possibly resulting from Ca 2+ influx through the NMDA receptors, results in SCOP truncation followed by ERK activation. In the consolidation period, m-calpain activation, possibly resulting from BDNF-mediated ERK activation [13] , stimulates mTOR-dependent protein synthesis through calpain-mediated PTEN degradation [14] , and in particular SCOP synthesis, which would restore normal SCOP levels, thereby preventing ERK activation. Full size image Our results also provide interesting information regarding the role of local protein synthesis in LTP. Although there is much debate regarding this issue with contradictory reports supporting or negating the requirement for protein synthesis [29] , [30] , our results indicate that at least during a short window of time following TBS, protein synthesis inhibition can enhance and not prevent LTP consolidation. This paradoxical effect of protein synthesis inhibition might have been easily missed, as the prevalent hypothesis is that protein synthesis is necessary for consolidation of LTP and memory. In particular, Cammalleri et al. [31] did not observe changes in LTP when they applied rapamycin after high-frequency stimulation. However, their stimulation protocol was very different from the one we used and could have produced LTP saturation. Our result also underscores the complexity of the function of local protein synthesis in LTP, and in learning and memory, and the critical role of the spatiotemporal sequence of events that are activated by TBS or by a learning experience. Protein homeostasis through synthesis and proteasome-mediated degradation has recently been proposed to play an important role in synaptic plasticity [26] . Our results indicate that calpain-mediated degradation is also an important contributor of protein homeostasis, as it provides a direct link between various extracellular signals, including glutamate and BDNF, with the local protein synthesis machinery regulated by the mTOR pathway. Previous studies had indicated that calpain-mediated SCOP degradation played a role in novel object recognition learning [6] , although the lack of effect of SCOP overexpression on fear conditioning suggested the possibility that different forms of learning and memory might use different types of signaling. Our results extend these findings and indicate that calpain-mediated SCOP regulation is more complex than previously reported, as calpain promotes both the degradation and synthesis of SCOP. The latter part of this duality provides a plausible explanation for recently discovered timing rules that obviate the normal limits on the magnitude of LTP. In particular, it has been reported that a second bout of theta burst stimulation does not produce additional LTP unless delivered after a delay of about 1 h, at which point it doubles the magnitude of potentiation [21] . It thus appears that induction and expression are followed by an extended refractory period. Additional work suggested that adult hippocampus contains a large population of spine synapses with high plasticity threshold, and that these are not driven into the potentiated state by a single episode of theta pattern stimulation [22] . Notably, the timing of the dual role of calpain in regulating SCOP metabolism matches that for the refractory period during which the high threshold synapses do not respond to a second train of theta bursts. If the two phenomena are closely related, then removing the calpain-mediated brake on LTP size should occlude the LTP2 effect. We confirmed this prediction by showing that a delayed theta train has no effect on the enhanced potentiation produced by a brief, post-TBS1 infusion of a calpain inhibitor. On the basis of the above, we propose that m-calpain-mediated increase of SCOP synthesis in the minutes following LTP depresses ERK activity at high threshold synapses, and thereby prevents them from transitioning into the potentiated state. The protease in this scenario serves to restrict single trial encoding of new information to a subset of synapses and imposes a delay before the initial representation can be expanded. It will be noted that this mechanism relates naturally to the distributed practice effect, a fundamental aspect of learning that has received little attention from neuroscientists. Specifically, training trials spaced apart by sizable delays produce much stronger memory than does a single, massed learning session [32] . The molecular brake described here may thus contribute importantly to the optimization of learning. It will be interesting to test whether m-calpain inhibitors enhance learning but do so at the cost of interfering with the spaced trials effect. In any event, our results provide a new description of the succession of events that take place following TBS in dendritic spines of field CA1 of the hippocampus ( Fig. 8 ). They place calpain activation at a central node of the various cascades of biochemical reactions that have been proposed to participate in the induction and consolidation stages of LTP [33] , [34] , in particular through the regulation of protein degradation and local protein synthesis of rapidly turning-over proteins, such as SCOP. Through this network, μ-calpain participates in LTP induction, whereas m-calpain limits the extent of synaptic enhancement, possibly by restricting the number of potentiated synapses to a subset of activated synapses. Superimposed on these cascades, calpain activation could also play important roles in the restructuring of the actin cytoskeleton and modification of the shape of dendritic spines, as we had proposed in our original hypothesis [7] . Thus, our findings provide a new framework to assemble the pieces of the complex events that are required to transform patterns of presynaptic activity in long-lasting changes in synaptic structure and function, and to explain certain temporal features of learning and memory. Acute hippocampal slice preparation Animal use in all experiments followed NIH guidelines and all protocols were approved by the Institution Animal Care and Use Committee of Western University of Health Sciences. Adult male Sprague–Dawley rats (3- to 4-month-old) were anaesthetized with halothane and decapitated. Brains were quickly removed and transferred to oxygenated, ice-cold cutting medium (in mM): 124 NaCl, 26 NaHCO 3 , 10 glucose, 3 KCl, 1.25 KH 2 PO 4 , 5 MgSO 4 and 3.4 CaCl 2 . Hippocampal transversal slices (400-μm-thick) were prepared using a McIlwain-type tissue chopper and transferred to either an interface recording chamber and exposed to a warm, humidified atmosphere of 95% O 2 /5% CO 2 and continuously perfused with oxygenated and preheated (33±0.5 °C) artificial cerebrospinal fluid (aCSF) (in mM: 110 NaCl, 5 KCl, 2.5 CaCl 2 , 1.5 MgSO 4 , 1.24 KH 2 PO 4 , 10 D -glucose, 27.4 NaHCO 3 ), perfused at 1.4 ml min −1 (electrophysiology); or a recovery chamber with a modified aCSF medium, containing (in mM): 124 NaCl, 2.5 KCl, 2.5 CaCl 2 , 1.5 MgSO 4 , 1.25 NaH 2 PO 4 , 24 NaHCO 3 , 10 D -glucose and saturated with 95% O 2 /5% CO 2 for 1 h at 37 °C (biochemical assays). CA1 minislices were obtained by dissecting out the CA1 region before transferring them in the recording chamber. Electrophysiology After 1.5 h incubation at 33±0.5 °C in the recording chamber, a single glass pipette filled with 2 M NaCl was used to record field excitatory postsynaptic potential elicited by stimulation of the Schaffer collateral pathway with twisted nichrome wires (single bare wire diameter, 50 μm) placed in CA1 stratum radiatum. Responses were recorded through a differential amplifier (DAM 50, World Precision Instruments, USA) with a 10-kHz high-pass and 0.1 Hz low-pass filter. Before each experiment, the input/output relation was examined by varying the intensity of the stimulation. Data were collected and digitized by Clampex, and the slope of field excitatory postsynaptic potential was analysed. All data are expressed as means±s.e.m., and statistical significance of differences between means was calculated with appropriate statistical tests as indicated in figure legends. Treatments of acute hippocampal slices After 1 h recovery, hippocampal slices were then transferred into screw-cap microfuge tubes containing 2 ml of freshly oxygenated aCSF medium with various drugs and were incubated at 37 °C for the indicated periods of times. For induction of chemical LTP, slices were transferred to a modified aCSF containing (in mM): NaCl (124), KCl (5), CaCl 2 (5), MgCl 2 (0.1), KH 2 PO 4 (1.25), NaHCO 3 (24), D -glucose (10) and TEA (25) for 10 min, and transferred back to normal aCSF. For calpain-inhibitor pretreatment, 10 μM CI-III (Calbiochem) was applied 15 min before changing the medium to the modified aCSF and during the incubation in modified aCSF. For calpain inhibitor post treatment, CI-III was applied 5 min after changing the medium back to normal aCSF. For BDNF treatment, slices were incubated in normal aCSF containing 100 ng ml −1 BDNF (Millipore) for the indicated time periods. For calpain-inhibitor pretreatment, CI-III was applied 15 min before application of BDNF. For calpain inhibitor post treatment, CI-III was applied 20 min after the application of BDNF. To inhibit protein synthesis, 25 μM cycloheximide (Tocris Bioscience) or 1 μM rapamycin (Cell Signaling) was applied 20 min before application of BDNF. At the indicated time points, two to three slices were rapidly frozen on dry ice. Slices were then lysed and protein concentrations were measured using BCA protein assay kit (Thermo). Equivalent amounts of proteins were processed for SDS–PAGE and western blotting. The primary antibodies used were SCOP (1:1,000, 07-1,341, Millipore), actin (1:10,000, MAB1501, Millipore), p-ERK (1:2,000, 9,101, Cell Signaling), ERK (1:3,000, 9,107) and Akt (1:1,500, 2,920). Full gel scans of all western blottings in this paper can be found in Supplementary Fig. 8 . Calpain assay The m-calpain-specific inhibitor, mCalp-I, was a generous gift from Dr James Power (Georgia Tech University). The hydrolysis of the fluorogenic substrate Suc-Leu-Tyr-AMC by μ-calpain and m-calpain was performed as previously described [35] , with minor modifications. Briefly, purified μ-calpain from porcine erythrocytes (8 μg, Millipore) or rat recombinant m-calpain (8 μg, a generous gift from Dr Peter Davis of Queen’s University, Ontario, Canada) was incubated with Suc-Leu-Tyr-AMC (0.5 mM) in 60 mM imidazole-HCl buffer, pH 7.3, containing 5 mM CaCl 2 , 5 mM cysteine, 2.5 mM β-mercaptoethanol and different concentrations of mCalp-I (ranging from 0 to 20 μM). The reaction was initiated by adding the enzyme and continued at 30 °C for 15 min, while the fluorescence of 7-amino-4-methylcoumarin (Ex 380 nm/Em 450 nm) was monitored every 30 s in a POLARstar Omega fluorescence polarization microplate reader (BMG Labtech). The rate of hydrolysis (increase in fluorescence per min) was determined from the linear portion of the curve. The IC 50 values were obtained by adjusting data from each experiment into a sigmoidal dose–response curve. The K i values for mCalp-I were calculated from the average of the IC 50 values and from a single substrate concentration by using a K i calculator tool for fluorescence-based competitive binding assays ( http://sw16.im.med.umich.edu/software/calc_ki/ ). The K m values of Suc-Leu-Tyr-AMC for μ-calpain and m-calpain are 4.74 and 2.21 mM, respectively [35] . The final concentrations for μ-calpain and m-calpain were 357 and 367 nM, respectively. Immunohistochemistry At the indicated time points after TBS, hippocampal slices were fixed in 4% paraformaldehyde for 1 h and cryoprotected in 30% sucrose for 1 h at 4 °C, and sectioned on a freezing microtome at 20 μm. Sections were blocked in 0.1 M PBS containing 10% goat serum and 0.4% Triton X-100, and then incubated in primary antibody mixture including rabbit anti-p-ERK (1:500, 4,370, Cell Signaling) and mouse anti-PSD-95 (1:500, MA1-045, Thermo) in 0.1 M PBS containing 5% goat serum and 0.4% Triton X-100 overnight at 4 °C. Sections were washed three times (10 min each) in PBS and incubated in Alexa Fluor 594 goat anti-rabbit IgG (A-11037, Life Technologies) and Alexa Fluor 488 goat anti-mouse IgG (A-11001) for 2 h at room temperature [36] . Cortical synaptoneurosome preparation Synaptoneurosomes were prepared from 3- to 4-month-old male Sprague–Dawley rats, as previously described [37] , with minor modifications. Briefly, cortices were rapidly dissected and placed into chilled modified Krebs solution containing (in mM): NaCl (118.5), KCl (4.7), KH 2 PO 4 (1.18), NaHCO 3 (24.9), MgSO 4 (1.18), CaCl 2 (2.5), D -glucose (10), HEPES (1), pH 7.4, and equilibrated with 95% O 2 /5% CO 2 . Cortices were homogenized in a 7-ml Kontes tissue Dounce homogenizer with ten strokes. Homogenized tissue was filtered through a 100-μm nylon mesh filter (BD Falcon) and the resulting suspension was filtered again through a 5-μm-pore size Acrodisc syringe filter with a Supor membrane (Pall Life Sciences). The filtrate was then centrifuged at 1,000 g for 15 min at 4 °C, washed once and centrifuged again. The pellet was resuspended in modified Krebs and drugs were directly added to the prewarmed (5 min, 37 °C) synaptoneurosome suspension for the indicated periods of time. Metabolic labelling of synaptoneurosomes and immunoprecipitation Detection of de novo protein synthesis was determined by using metabolic labelling with Click-iT L -azidohomoalanine (AHA, Molecular Probes). Cortical synaptoneurosomes were pre-incubated with 500 μM AHA in the absence and presence of 1 μM rapamycin for 20 min, and then treated with 100 ng ml −1 of BDNF for 60 min. After washing out the treatments, samples were incubated with phosphine-PEG3-Biotin (Thermo) for 4 h at 37 °C, to conjugate biotin to AHA-containing proteins. Samples were then eluted on Zeba Spin desalting columns (7K MWCO, Thermo) to remove the excess of phosphine-PEG3-Biotin. Equal amount of proteins (~5 mg ml −1 ) were incubated with SCOP antibody (1:100, Bethyl Laboratories) overnight at 4 °C. Subsequently, 50 μl of protein A-sepharose beads (1:1 slurry, Sigma) were added to each sample and incubated for 1 h at 4 °C with gentle rocking. After three washes, samples were processed for SDS–PAGE and western blotting. IRDye 800CW Streptavidin (1:2,000, LI-COR Biosciences) was used to detect biotin-conjugated (newly synthesized) SCOP. Anti-SCOP antibody (1:1,000, Millipore) was used to detect total immunoprecipitated SCOP. Statistical analyses For LTP experiments where only two groups were compared, we used the two-tail t -test for determining statistical significance. When more than two groups were compared, we used one-way analysis of variance followed by Bonferroni test to determine statistical significance. For the analyses of time-dependent change of SCOP, PTEN and p-ERK after various treatments, the ratios of SCOP to Akt (loading control), PTEN to Akt and phospho-ERK 1/2 to total ERK 1/2 were compared at different time points. All values were divided by the average value at time point 0 for normalization. Comparison with time point 0 was performed by one-way analysis of variance followed by Bonferroni test. How to cite this article: Wang, Y. et al. A molecular brake controls the magnitude of long-term potentiation. Nat. Commun. 5:3051 doi: 10.1038/ncomms4051 (2014).